RETRACTED ARTICLE: The association between early career informal mentorship in academic collaborations and junior author performance We study mentorship in scientific collaborations, where a junior scientist is supported by potentially multiple senior collaborators, without them necessarily having formal supervisory roles. We identify 3 million mentor–protégé pairs and survey a random sample, verifying that their relationship involved some form of mentorship. We find that mentorship quality predicts the scientific impact of the papers written by protégés post mentorship without their mentors. We also find that increasing the proportion of female mentors is associated not only with a reduction in post-mentorship impact of female protégés, but also a reduction in the gain of female mentors. While current diversity policies encourage same-gender mentorships to retain women in academia, our findings raise the possibility that opposite-gender mentorship may actually increase the impact of women who pursue a scientific career. These findings add a new perspective to the policy debate on how to best elevate the status of women in science. Mentorship contributes to the advancement of individual careers [1] , [2] , [3] and provides continuity in organizations [4] , [5] . By mentoring novices, senior members pass on the organizational culture, best practices, and the inner workings of a profession. In this way, the mentor–protégé relationship provides the social glue that links generations within a field. Mentorship can also alleviate the barriers of entry for underrepresented minorities, such as women and people of color by providing role models, access to informal networks and cultural capital, thereby acting as an equalizing force [6] , [7] , [8] , [9] , [10] . Most workplaces have shifted from the classic master-apprentice model towards a team-based model, where the mentorship of juniors is distributed amongst the senior members of the team. As a result, it has become commonplace for juniors to be mentored by senior colleagues, without them necessarily being their formal supervisors [11] , [12] . In the context of academic collaboration, the role of mentorship in supporting early-career scientists is widely recognized [13] . We analyze mentorship in this context, where a less experienced scientist is mentored by more experienced collaborators, without restricting our analysis to only the thesis advisor. Academic publications provide a documented record of millions of collaborations spread over decades, and have already proven to be a fertile ground for exploring a wide variety of topics, including innovation [14] , diversity [15] , productivity [16] , team assembly [17] , [18] , and individual success [19] , [20] , [21] , thereby giving rise to the field of Science of Science [22] . We harness the potential of this rich dataset to study mentorship by analyzing academic collaborations between junior and senior scientists, since such collaborations play an important role in shaping the junior scientist’s persona, both in terms of their research focus [23] , professional ethics, and work culture [24] . Furthermore, we build on the expanding literature on gender equity and diversity in science [25] , [26] , [27] , [28] , [29] , [30] and analyze the mentorship experiences from the perspective of both female and male scientists. Compared to previous studies on mentorship in academia [31] , [32] , [33] , [34] , [35] , [36] , [37] , [38] , ours has the following advantages. First, instead of restricting our analysis to the thesis advisor, we study mentorship in its broader sense, which may involve multiple senior collaborators who may or may not hold a formal supervisory role. Second, we avoid sample selectivity as well as recall and recency biases, since we analyze the actual scientific impact of collaborations rather than self-reported information. Third, we analyze thousands of journals spanning multiple scientific disciplines, rather than restricting our focus to just a single one of them. Fourth, we construct careful comparisons between millions of mentor–protégé pairs, allowing us to better understand the association between mentorship quality and scientific careers. Finally, our study complements the literature on the relationship between mentorship and attrition from science [39] , as we consider protégés who remain scientifically active after the completion of their mentorship period. It should be noted that we are not the first to study how the impact of junior scientists is related to the impact of their past collaborators. A recent study by Li et al. [40] found that juniors who publish with top scientists enjoy a persistent competitive advantage throughout the rest of their careers. More specifically, they focus on collaborators who are among the 5% most impactful scientists in any given year, regardless of whether they are senior or junior. In contrast, as we will show, our study focuses on collaborators who are likely to have served as mentors, regardless of whether they are among the top 5%. In other words, Li et al. study coauthorship with top scientists, while we study coauthorship with mentors. Another difference between their study and ours is that they do not address the fundamental question of whether the social capital of collaborators matters more than their impact; we address this question by analyzing not only the mentors’ impact but also their collaboration network. Finally, unlike their paper, our study complements existing literature on women in science, by analyzing the gender of both the protégés and their mentors, and how these shape mentorship experiences. Another recent paper that is closely related to ours is the one by Ma et al. [41] , who study how the success of junior scientists is related to the ability of their mentors to create and communicate prizewinning research. As such, their work resembles ours in the sense that they also study some form of academic success and how it is related to mentorship. However, they study formal mentorship, where the mentor is the official PhD advisor of the protégé. In contrast, our study covers informal mentorship whereby juniors are mentored by multiple senior colleagues without them necessarily having formal supervisory roles. Furthermore, their analysis of the protégé’s performance post mentorship includes papers written with the mentors, leading to their finding that coauthoring with one’s advisor is inversely correlated with one’s success. In contrast, our analysis excludes papers written with any of the scientists who served as mentors during the mentorship experience; this ensures that the observed impact is not attributed to the mentors but rather to the protégés. Identifying mentor–protégé pairs We analyze 215 million scientists and 222 million papers taken from the Microsoft Academic Graph (MAG) dataset [42] , which contains detailed records of scientific publications and their citation network. We address the name disambiguation problem (see Supplementary Note 1 ), and we use other external data-generating techniques and sources to establish the gender of scientists and the rank of their affiliations (see “Methods” section and Supplementary Note 2 ). We distinguish between junior and senior scientists based on their academic age, measured by the number of years since their first publication. The junior years are those during which a scientist participates in graduate and postdoctoral training, and possibly the first few years of being a faculty member or researcher. In contrast, the senior years are those during which a scientist typically accumulates experience as a PI and transitions into a supervisory role. For any given scientist, we consider the first 7 years of their career to be their junior years, and the ones after that to be their senior years. Whenever a junior scientist publishes a paper with a senior scientist, we consider the former to be a protégé, and the latter to be a mentor, as long as they coauthored at least one paper with 20 or less co-authors and share the same discipline and US-based affiliation; see Supplementary Note 3 for more details. Our use sample consists of 3 million unique mentor–protégé pairs, spanning ten disciplines (Biology, Chemistry, Computer Science, Economics, Engineering, Geology, Materials Science, Medicine, Physics, and Psychology) and over a century of research; these disciplines contain over 97% of all pairs identified as per the criteria above. Survey results While we acknowledge that it is possible for juniors to receive support from their junior collaborators, we interpret mentorship as the support that juniors receive from their senior collaborators, following the standard definition of mentorship as “the activity of giving a younger or less experienced person help and advice over a period of time” https://dictionary.cambridge.org/dictionary/english/mentorship . Based on this definition, the difference in experience between the protégé and their mentor seems to be a necessary, albeit not sufficient, condition for the relationship to be considered mentorship. In addition to the difference in experience, the relationship also needs to involve some form of support from the mentor to the protégé. Arguably, the fact that the mentor has coauthored a paper with the protégé provides evidence that the former indeed supported the latter. Nevertheless, it would be desirable to provide further evidence that the mentor supported the protégé in ways related not only to the paper on which they are collaborating, but also to career development in general. To verify whether this is the case, we sampled 2000 scientists whom we identified as protégés, to ask them about their relationship with their mentors. We manually extracted their emails from publicly available sources, such as their personal web pages, and invited them to fill out a survey about scientific collaborations. Out of those 2000 scientists, 167 completed the survey; see Supplementary Note 4 for more details. A summary of the survey results is provided in Fig. 1 . More specifically, Fig. 1 a presents the distribution of the responses to five questions, each asking whether the protégé has received advice from the mentor about a different career-building skill. As can be seen, for each skill, a high percentage of protégés agreed (strongly or otherwise) that they have received advice from the senior collaborator about that skill, with the percentage ranging from 72 to 85% depending on the skill. Fig. 1: Survey outcome. Responses of 167 randomly-chosen scientists who were identified as protégés and asked about their relationship to a scientist who was identified as one of their mentors. a Distributions of the responses to each of five statements regarding their senior collaborator, where the statements take the form “I received advice from him/her about...” followed by five different skills: (i) writing; (ii) research study/design; (iii) data analysis/modeling; (iv) addressing reviewer comments; (v) selecting a venue for publication. b A different way of summarizing the responses in a , showing the proportion of participants who either agree or strongly agree to at least x out of the five statements regarding their senior collaborator, where x ∈ {1, …, 5}. c The percentage of protégés who selected true for each of the following four statements regarding their senior collaborator: (i) I received grant writing advice from him/her; (ii) I received a letter of recommendation from him/her for a fellowship/award or job application; (iii) I received career planning advice from him/her; (iv) He/she put me in touch with an important person in my field. d A different way of summarizing the responses in c , showing the proportion of participants who have selected true to at least x out of the four statements regarding their senior collaborator, where x ∈ {1, …, 4}. Source data are provided as a Source Data file. 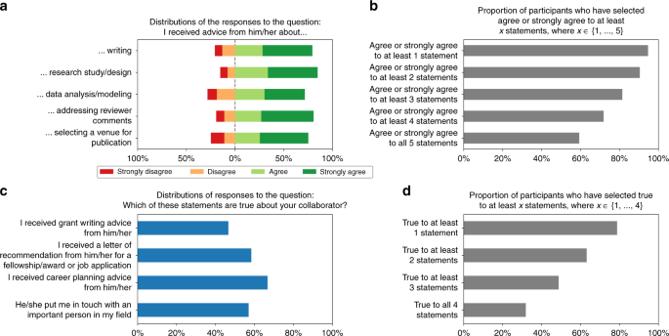Fig. 1: Survey outcome. Responses of 167 randomly-chosen scientists who were identified as protégés and asked about their relationship to a scientist who was identified as one of their mentors.aDistributions of the responses to each of five statements regarding their senior collaborator, where the statements take the form “I received advice from him/her about...” followed by five different skills: (i) writing; (ii) research study/design; (iii) data analysis/modeling; (iv) addressing reviewer comments; (v) selecting a venue for publication.bA different way of summarizing the responses ina, showing the proportion of participants who either agree or strongly agree to at leastxout of the five statements regarding their senior collaborator, wherex∈{1, …, 5}.cThe percentage of protégés who selected true for each of the following four statements regarding their senior collaborator: (i) I received grant writing advice from him/her; (ii) I received a letter of recommendation from him/her for a fellowship/award or job application; (iii) I received career planning advice from him/her; (iv) He/she put me in touch with an important person in my field.dA different way of summarizing the responses inc, showing the proportion of participants who have selected true to at leastxout of the four statements regarding their senior collaborator, wherex∈{1, …, 4}. Source data are provided as a Source Data file. Full size image Figure 1 b summarizes the responses differently, by presenting the percentage of protégés who agreed (strongly or otherwise) to at least x out of the five skills, where x ranges from 1 to 5. As can be seen, 95% agreed (strongly or otherwise) that they have received advice from their senior collaborator regarding at least one skill. Figure 1 c, d summarize the responses to a different set of questions, focusing on the support that the protégé has received from the senior collaborator regarding different aspects of career development, outside the context of their joint publication. We find that almost 80% have stated that they have received advice from their senior collaborator regarding at least one of those aspects. Similar trends were observed when considering only the protégés who stated that the identified mentor was not their thesis advisor nor a member of their thesis committee; see Supplementary Fig. 1 . Broadly similar trends were also observed when considering each discipline in isolation; see Supplementary Figs. 2 – 5 . Altogether, these findings indicate that the relationship between our identified protégés and mentors indeed involved some form of mentorship. Analyzing mentor–protégé pairs When analyzing all our mentor–protégé pairs, we consider two alternative measures of mentorship quality. The first is the average impact of the mentors prior to mentorship, where the prior impact of each mentor is computed as their average number of citations per annum up to the year of their first publication with the protégé. This reflects the success of mentors and their standing and reputation in their respective scientific communities. We refer to this measure as the big-shot experience, as it captures how much of a “big-shot” the mentors of the protégé are. The second measure of mentorship quality that we consider is the average degree of the mentors prior to mentorship, where the degree of each mentor is calculated in the network of scientific collaborations up to the year of their first publication with the protégé [43] , [44] . We refer to this measure as the hub experience, as it reflects how much of a “hub” each mentor is in the collaboration network. These two measures of mentorship experience take the role of independent variables in our study. Having discussed our measures of mentorship quality, we now discuss the mentorship outcome, which we conceptualize as the scientific impact of the protégé during their senior years without their mentors. We measure this outcome by calculating the average impact of all the papers that satisfy the following two conditions: (i) they were published when the academic age of the protégé was greater than 7 years; (ii) the authors include the protégé but none of the scientists who were identified as their mentors. The impact of each such paper is calculated as the number of citations that it accumulated 5 years post publication, denoted by c 5 [15] ; this is the measure of scientific impact that will be used throughout the article. Such an outcome measure allows us to assess the quality of the scholar that the protégé has become after the mentorship period has concluded. We aim to establish whether mentorship quality (measured by big-shot experience or network experience) is associated with the post-mentorship outcome. To this end, we use coarsened exact matching (CEM) [45] . While this technique does not establish the existence of a causal effect, it is commonly used to infer causality from observational data. Intuitively, CEM allows us to select a group of protégés who received a certain level of mentorship quality (treatment group), and match it to another group of protégés who received a lower level of mentorship quality (control group). Comparing the outcome of the two groups allows us to determine whether an increase in mentorship quality is indeed associated with an increase in the impact of the protégé post mentorship. In more detail, for each measure of mentorship quality, we create a separate CEM where the treatment and control groups differ in terms of that measure, but resemble each other in terms of an array of characteristics of the protégés, in particular, the number of mentors they have, the year in which they published their first mentored paper, their scientific discipline, their gender, the rank of the affiliation listed on their first mentored publication (which is likely to be their PhD granting institution), the number of years active post mentorship, and the average academic age of their mentors, which is measured by first computing the academic age of each mentor in the year of their first publication with the protégé, and then averaging these numbers over all the mentors. Importantly, when studying the big-shot experience, we make sure that the two groups are also similar in terms of the hub experience, and vice versa. For every independent variable, be it big-shot experience or hub experience, let Q i denote the i th quintile of the distribution of that variable. Then, for i ∈ {1, 2, 3, 4}, we build a separate CEM where the treatment and control groups are Q i +1 and Q i , respectively. The CEM results are depicted in Fig. 2 . These results indicate that an increase in big-shot experience is significantly associated with an increase in the post-mentorship impact of protégés by up to 35%. Similarly, the hub experience is associated with an increase the post-mentorship impact of protégés, although the increase never exceeds 13%. Furthermore, our analysis in Supplementary Note 5.3 and Supplementary Figs. 6 , 7 suggests that these observations are not driven by differences in the protégés’ innate ability. Fig. 2: The big-shot experience and hub experience of 3 million mentor–protégé pairs. For every independent variable, be it big-shot experience or hub experience, Q i denotes the i th quintile of the distribution of that variable. For i ∈ {1, 2, 3, 4}, we consider Q i +1 and Q i to be the treatment and control groups, respectively, and write Q i +1 vs. Q i when referring to the CEM used to compare these two groups. The color of the bar indicates whether the independent variable is the big-shot experience (purple) or the hub experience (yellow), whereas the height of the bar equals δ , which is the increase in the average post-mentorship impact of the treatment group relative to that of the control group. A t -test shows that the values of δ are all statistically significant; see the corresponding p -values in Supplementary Tables 2 and 3 . Since scientific impact is sensitive to external values, we bootstrap a 95% confidence interval. The error bars represent the 95% confidence interval. *** p < 0.001, ** p < 0.01, * p < 0.05. Source data are provided as a Source Data file. Full size image Next, we compare the big-shot experience to the hub experience. As can be seen in Fig. 2 , the mentorship outcome seems to be much more strongly associated with big-shot experience than with the hub experience. Supplementary Figs. 8 – 12 as well as Supplementary Tables 8 – 17 show similar trends when (i) replacing c 5 with c 10 as per Sinatra et al. [46] ; (ii) computing our measures of mentorship quality using the maximum and median values instead of the average value; (iii) considering juniors and seniors to be those whose academic age is at most 6 and at least 9, respectively; and (iv) considering juniors and seniors to be those whose academic age is at most 5 and at least 10, respectively. Similar trends would also be observed if we replace the average with the sum in our measures of mentorship quality, since we are controlling for the number of mentors; see Supplementary Note 5.1 for more details. These findings imply that the scientific impact of the mentors matters more than their number of collaborators. Consequently, we restrict our attention to the big-shot experience throughout the remainder of our study. Supplementary Figs. 13 – 18 as well as Supplementary Tables 18 – 23 suggest that the association between big-shot experience and mentorship outcome persists regardless of the discipline, the affiliation rank, the number of mentors, the average age of the mentors, the protégé’s gender, and the protégé’s first year of publication. The relationship between gender and mentorship Next, we turn to a different exploratory analysis where we investigate the post-mentorship impact of protégés while taking into consideration their gender as well as the gender of their mentors. To this end, let F i denote the set of protégés that have exactly i female mentors. We take the protégés in F 0 as our baseline, and match them to those in F i for i ∈ {1, 2, 3, 4, 5}, while controlling for the protégé’s average big-shot experience, number of mentors, gender, discipline, affiliation rank, and the year in which they published their first mentored paper. Then, we vary the fraction of female mentors to understand how this affects the protégé. More specifically, for any given i > 0, we compute the change in the post-mentorship impact of the protégés in F i relative to the post-mentorship impact of those in F 0 , which we refer to by writing F i vs. F 0 . The outcomes of these comparisons are depicted for male protégés in Fig. 3 a, and for female protégés in Fig. 3 b. As shown in this figure, having more female mentors is associated with a decrease in the mentorship outcome, and this decrease can reach as high as 35%, depending on the number of mentors and the proportion of female mentors. Fig. 3: The relationship between gender and the gain from mentorship. a F i denotes the set of protégés from our 3 million pairs that have exactly i female mentors. Focusing on male protégés, F i vs. F 0 : i = 1, …, 5 refers to the change in the average post-mentorship impact of protégés in F i relative to the average post-mentorship impact of those in F 0 while controlling for the protégé’s big-shot experience, number of mentors, discipline, affiliation rank, and the year in which they published their first mentored paper. 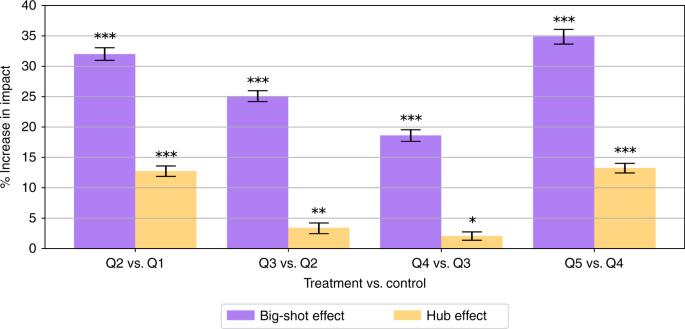Fig. 2: The big-shot experience and hub experience of 3 million mentor–protégé pairs. For every independent variable, be it big-shot experience or hub experience,Qidenotes theith quintile of the distribution of that variable. Fori∈{1, 2, 3, 4}, we considerQi+1andQito be the treatment and control groups, respectively, and writeQi+1vs.Qiwhen referring to the CEM used to compare these two groups. The color of the bar indicates whether the independent variable is the big-shot experience (purple) or the hub experience (yellow), whereas the height of the bar equalsδ, which is the increase in the average post-mentorship impact of the treatment group relative to that of the control group. At-test shows that the values ofδare all statistically significant; see the correspondingp-values in Supplementary Tables2and3. Since scientific impact is sensitive to external values, we bootstrap a 95% confidence interval. The error bars represent the 95% confidence interval. ***p< 0.001, **p< 0.01, *p< 0.05. Source data are provided as a Source Data file. 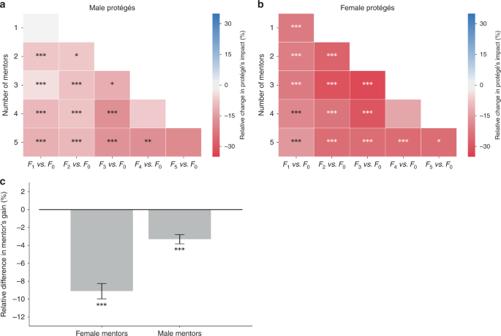Fig. 3: The relationship between gender and the gain from mentorship. aFidenotes the set of protégés from our 3 million pairs that have exactlyifemale mentors. Focusing on male protégés,Fivs.F0:i= 1, …, 5 refers to the change in the average post-mentorship impact of protégés inFirelative to the average post-mentorship impact of those inF0while controlling for the protégé’s big-shot experience, number of mentors, discipline, affiliation rank, and the year in which they published their first mentored paper. A t-test is used to show the that values are all satistically significant; see the correspondingp-values in Supplementary Table24.bThe same asabut for female protégés instead of male protégés.cThe gain of a mentor when mentoring a particular protégé is measured as the average impact (〈c5〉) of the papers they authored with that protégé during the mentorship period. While controlling for the protégé’s discipline, affiliation rank, number of mentors, and the year in which they published their first mentored paper, the figure depicts the change in the mentor’s average gain when mentoring a female protégé relative to that when mentoring a male protégé; results are presented for female mentors and male mentors separately. At-test shows that the values are all statistically significant. Since scientific impact is sensitive to external values, we bootstrap a 95% confidence interval. The error bars represent the 95% confidence interval. *p< 0.05, **p< 0.01, ***p< 0.001. Source data are provided as a Source Data file. A t-test is used to show the that values are all satistically significant; see the corresponding p -values in Supplementary Table 24 . b The same as a but for female protégés instead of male protégés. c The gain of a mentor when mentoring a particular protégé is measured as the average impact (〈 c 5 〉) of the papers they authored with that protégé during the mentorship period. While controlling for the protégé’s discipline, affiliation rank, number of mentors, and the year in which they published their first mentored paper, the figure depicts the change in the mentor’s average gain when mentoring a female protégé relative to that when mentoring a male protégé; results are presented for female mentors and male mentors separately. A t -test shows that the values are all statistically significant. Since scientific impact is sensitive to external values, we bootstrap a 95% confidence interval. The error bars represent the 95% confidence interval. * p < 0.05, ** p < 0.01, *** p < 0.001. Source data are provided as a Source Data file. Full size image So far in our analysis, we only considered the outcome of the protégés. However, mentors have also been shown to benefit from the mentorship experience [1] . With this in mind, we measure the gain of a mentor from a particular protégé as the average impact, 〈 c 5 〉, of the papers they authored with that protégé during the mentorship period. We compare the average gain of a female mentor, F , against that of a male mentor, M , when mentoring either a female protégé, f , or a male protégé, m . More specifically, we compare mentor–protégé relationships of the type ( f , F ) to those of the type ( m , F ), where f and m are matched based on their discipline, affiliation rank, number of mentors, and the year in which they published their first mentored paper. Similarly, we compare relationships of the type ( f , M ) to those of the type ( m , M ), where f and m are matched as above. The results of these comparisons are presented in Fig. 3 c. In particular, the figure depicts the gain from mentoring a female protégé relative to that of mentoring a male protégé; the results are presented for female mentors and male mentors, separately. These results suggest that, by mentoring female instead of male protégés, the female mentors compromise their gain from mentorship, and suffer on average a loss of 18% in citations on their mentored papers. As for male mentors, their gain does not appear to be significantly affected by taking female instead of male protégés. In this paper, we studied mentorship in academic collaborations, where junior scientists receive support from potentially multiple senior collaborators without necessarily having a formal supervisory role. We identified 3 million mentor–protégé pairs, and conducted a survey with a random sample of protégés, the outcome of which provided evidence that the relationship between them and their identified mentors involved some form of mentorship. Furthermore, having conceptualized mentorship quality in two ways—the big-shot experience and the hub experience—we found that both have an independent association with the protégé’s impact post mentorship without their mentors. Interestingly, the big-shot experience seems to matter more than the hub experience, implying that the scientific impact of mentors matters more than the number of their collaborators. Our analysis also suggests that the association between the big-shot experience and the post-mentorship outcome persists regardless of the discipline, the affiliation rank, the number of mentors, the average age of the mentors, the protégé’s gender, and the protégé’s first year of publication. Finally, we studied the possibility that the gender of both the mentors and their protégé could predict not only the impact of the protégé, but also the gain of the mentors, which we measure by the citations of the papers they published with the protégé during the mentorship period. Future research could investigate the mechanisms that underlie our findings, e.g., (i) by comparing mentors who are newcomers to those who are incumbents [17] , (ii) by analyzing the papers that cite the protégés to see how many of those are authored by the mentors’ collaborators, and (iii) by studying the topics that the protégés work on during, and after, the mentorship to understand the skills that are transferred from the mentors to their protégés. These would be welcome extensions to the study, but remain outside of its current scope. While it has been shown that having female mentors increases the likelihood of female protégés staying in academia [10] and provides them with better career outcomes [39] , such studies often compare protégés that have a female mentor to those who do not have a mentor at all, rather than to those who have a male mentor. Our study fills this gap, and suggests that female protégés who remain in academia reap more benefits when mentored by males rather than equally-impactful females. The specific drivers underlying this empirical fact could be multifold, such as female mentors serving on more committees, thereby reducing the time they are able to invest in their protégés [47] , or women taking on less recognized topics that their protégés emulate [48] , [49] , [50] , but these potential drivers are out of the scope of current study. Our findings also suggest that mentors benefit more when working with male protégés rather than working with comparable female protégés, especially if the mentor is female. These conclusions are all deduced from careful comparisons between protégés who published their first mentored paper in the same discipline, in the same cohort, and at the very same institution. Having said that, it should be noted that there are societal aspects that are not captured by our observational data, and the specific mechanisms behind these findings are yet to be uncovered. One potential explanation could be that, historically, male scientists had enjoyed more privileges and access to resources than their female counterparts, and thus were able to provide more support to their protégés. Alternatively, these findings may be attributed to sorting mechanisms within programs based on the quality of protégés and the gender of mentors. Our gender-related findings suggest that current diversity policies promoting female–female mentorships, as well-intended as they may be, could hinder the careers of women who remain in academia in unexpected ways. Female scientists, in fact, may benefit from opposite-gender mentorships in terms of their publication potential and impact throughout their post-mentorship careers. Policy makers should thus revisit first and second order consequences of diversity policies while focusing not only on retaining women in science, but also on maximizing their long-term scientific impact. More broadly, the goal of gender equity in science, regardless of the objective targeted, cannot, and should not be shouldered by senior female scientists alone, rather, it should be embraced by the scientific community as a whole. Data description The data used for this study consists of all the papers included in the Microsoft Academic Graph (MAG) dataset up to December 31st, 2019 [42] , [51] . This dataset includes records of scientific publications specifying the date of the publication, the authors’ names and affiliations, and the publication venue. It also contains a citation network in which every node represents a paper and every directed edge represents a citation. While the number of citations of any given paper is not provided explicitly, it can be calculated from the citation network in any given year. Additionally, every paper is positioned in a field-of-study hierarchy, the highest level of which is comprised of 19 scientific disciplines. Using the information provided in the MAG dataset, we derive two key measures: the discipline of scientists and their impact. In particular, to determine the discipline of any given scientist, we consider his or her publications, which are themselves classified into disciplines by MAG. If 50% or more of those papers were from the same discipline, d i , then the scientist’s discipline is considered to be d i ; otherwise it is considered to be unclassified. As for the impact of each scientist in any given year, it was derived from the citation network provided by MAG. In addition to the scientists’ discipline and impact, we derive additional measures such as the scientists’ gender, which is determined using Genderize.io [52] (see Supplementary Note 2 ), and the rank of each university, which is determined based on the Academic Ranking of World Universities, also known as the Shanghai ranking http://www.shanghairanking.com/ARWU2018.html . Whenever a junior scientist (with academic age ≤ 7) publishes a paper with a senior scientist (academic age  > 7), we consider the former to be a protégé, and the latter to be a mentor. We consider the start of the mentorship period to be the year of the first publication of the protégé, and consider the end of the mentorship period to be the year in which the protégé became a senior scientist. We analyze every mentor–protégé dyad that satisfies all of the following conditions: (i) the protégé has at least one publication during their senior years without a mentor; (ii) the affiliation of the protégé is in the US throughout their mentorship years; (iii) the main discipline of the mentor is the same as that of the protégé; (iv) the mentor and the protégé share an affiliation on at least one publication; (v) during the mentorship period, the mentor and the protégé worked together on a paper whose number of authors is 20 or less; and (vi) the protégé does not have a gap of 5-years or more in their publication history. As a consequence, our analysis excludes all scientists: (i) who never published any papers without their mentors post-mentorship, as we cannot analyze their scientific impact in their senior years independent of their mentors; (ii) who only had solo-authored papers or collaborations with their junior peers or with seniors from other universities, as we cannot clearly establish who their mentors were; (iii) who had a gap longer than 5-years without any publications; and (iv) who only collaborated with senior scientists outside of their main discipline. As our use sample we consider the ten disciplines in MAG that have the largest number of mentor–protégé pairs, namely Biology, Chemistry, Computer Science, Economics, Engineering, Geology, Materials Science, Medicine, Physics, and Psychology. These disciplines contain over 97% of all pairs identified as per the criteria above; see Supplementary Table 1 . A total of 204 different Coarsened Exact Matchings (CEMs) were used to produce the results depicted in Fig. 2 and Supplementary Figs. 6 – 18 . Additionally, a total of 32 different matchings were used to produce the results depicted in Fig. 3 . More details about the confounding factors used therein, as well as the binning decisions, can all be found in the Supplementary Note 5.1 . Ethics statement The survey portion of the study was approved by the NYUAD Institutional Review Board, #HRPP-2020-8. Informed consent was obtained from all of the participants, who also received incentives. Reporting summary Further information on research design is available in the Nature Research Reporting Summary linked to this article.